Fork sensing and strand switching control antagonistic activities of RecQ helicases RecQ helicases have essential roles in maintaining genome stability during replication and in controlling double-strand break repair by homologous recombination. Little is known about how the different RecQ helicases found in higher eukaryotes achieve their specialized and partially opposing functions. Here, we investigate the DNA unwinding of RecQ helicases from Arabidopsis thaliana , AtRECQ2 and AtRECQ3 at the single-molecule level using magnetic tweezers. Although AtRECQ2 predominantly unwinds forked DNA substrates in a highly repetitive fashion, AtRECQ3 prefers to rewind, that is, to close preopened DNA forks. For both enzymes, this process is controlled by frequent strand switches and active sensing of the unwinding fork. The relative extent of the strand switches towards unwinding or towards rewinding determines the predominant direction of the enzyme. Our results provide a simple explanation for how different biological activities can be achieved by rather similar members of the RecQ family. RecQ helicases are involved in different steps of DNA structure processing that arise, for example, during DNA replication, telomere maintenance, DNA repair and DNA recombination [1] , [2] , [3] . The proteins belong to the SF2 family of helicases and have a 3′–5′ directionality. In humans, mutations in the corresponding RecQ genes can lead to severe genetic disorders like Werner syndrome (WRN affected), Bloom’s syndrome (BLM affected) and Rothmund–Thomson syndrome (RECQ4 affected). RecQ helicases are conserved within all kingdoms of life with the tendency that multicellular organisms possess several homologues, for example, five in humans and seven in the model plant Arabidopsis thaliana [4] . The presence of multiple RecQ helicases in the same organism strongly indicates sub- or neo-functionalization during the evolution of this gene family. Some of the functions of paralogous RecQ helicases may overlap, but mostly, the enzymes have specialized functions, which is also reflected by the fact that different diseases are caused by mutations of different human RecQ helicases. Up to now, however, it remains unclear how this specialization is accomplished at the molecular level. For example, two proteins with a high level of sequence similarity can have opposing functions in vivo : Mutants of the RecQ member AtRECQ4A show hyper-recombination and sensitivity against DNA-damaging agents, whereas for AtRECQ4B mutants hypo-recombination and no sensitivity was reported despite 70% sequence identity [5] , [6] . To address the question how different RecQ helicases may achieve their dedicated function, we investigate here the DNA unwinding of two RecQ helicases from A. thaliana —RECQ2, the probable functional homologue of the WRN protein in humans [7] and RECQ3 (ref. 8 ). For this, we use single-molecule measurements that have in recent years become a valuable complement to X-ray crystallography and classical biochemical methodology in mechanistic investigations of helicases. They have, for example, helped to directly measure DNA unwinding, single-strand DNA (ssDNA) and double-strand DNA (dsDNA) translocation velocities, enabled determination of the forward stepping of helicases on DNA and provided insight into the activeness of the unwinding [9] , [10] , [11] , [12] . Most importantly, they revealed the partially rich dynamics of (re)initiation and termination of the DNA translocation/unwinding process [13] , [14] , [15] . Using single-molecule FRET measurements, for example, the human RecQ helicase BLM was found to unwind only a limited number of base pairs (bp), then to return and to reinitiate new unwinding events in a highly repetitive fashion [16] . Such highly repetitive unwinding events have been thought to be important for biological functions, for example, to process stalled replication forks, eliminate potentially deleterious recombination intermediates or as observed for ssDNA translocases, to strip off other DNA-binding proteins [16] , [17] , [18] . Using magnetic tweezers that allow the following of DNA unwinding in real-time with 2–3 bp resolution, we find here that the related RecQ helicases AtRECQ2 and AtRECQ3 both show highly repetitive DNA unwinding, suggesting that this is a general feature of RecQ helicases. The repetitive events are driven by frequent strand switches, which allow the enzymes to place themselves in a favored orientation with respect to the fork. Although AtRECQ2 preferentially orients itself towards the junction to unwind it, AtRECQ3 moves in the opposite direction and processively rewinds, that is, helps closing, unzipped hairpins over hundreds of bases. This shows that RecQ helicases can exhibit antagonistic activities on the molecular level and provides mechanistic insight into how very different cellular activities may be accomplished by closely related enzymes. Repetitive DNA unwinding by single AtRECQ2 enzyme complexes To study DNA unwinding by AtRECQ2 at the single-molecule level we use magnetic tweezers [19] . For this, a DNA substrate is prepared that consists of a 40 base pairs (bp) long DNA hairpin with a three-nucleotide (nt) end-loop ( Supplementary Fig. S1a ). The hairpin is attached at its 5′-end to a magnetic bead and at its 3′-end through a 44 nt ssDNA initiation site for the helicase and a 600-bp long dsDNA spacer to the surface of the fluidic cell of the setup. Using a pair of magnets, the hairpin ends are stretched and simultaneously the ssDNA length of the hairpin is determined. The hairpin can be mechanically unzipped by applying forces larger than the critical force F unzip for which the 40 bp of the hairpin open in one fast event, which is seen as an abrupt length change of the expected size of 38 nm corresponding to 83 nt ( Fig. 1a ). 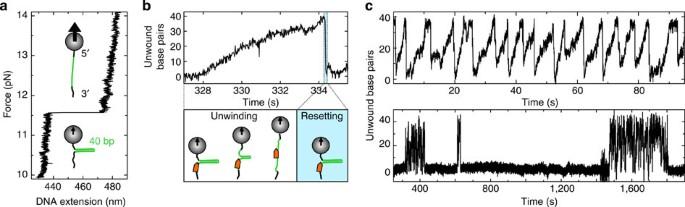Figure 1: DNA hairpin unwinding by AtRECQ2. (a) Force induced hairpin unzipping. Increasing the force applied to the hairpin construct (seeSupplementary Fig. S1b) leads initially to slight stretching of the dsDNA handles of the construct. At a critical force (Funzip=11.6 pN) the 40 bp long hairpin unzips in a single abrupt step followed by further slight extension increases. (b) Typical unwinding event of AtRECQ2 on a 40 bp hairpin in the presence of ATP at a constant force of 10 pN. After slow hairpin unwinding an abrupt rezipping of the hairpin occurs followed by a resetting, that is, the reinititation of a new unwinding event (see sketches below). (c) Global unwinding pattern of AtRECQ2 on the 40 bp DNA hairpin under the same conditions as inb. (upper) Individual saw tooth-like events of similar size occur in a highly repetitive fashion. (lower). Periods of highly repetitive unwinding events are interspersed with periods of no activity. Figure 1: DNA hairpin unwinding by AtRECQ2. ( a ) Force induced hairpin unzipping. Increasing the force applied to the hairpin construct (see Supplementary Fig. S1b ) leads initially to slight stretching of the dsDNA handles of the construct. At a critical force ( F unzip =11.6 pN) the 40 bp long hairpin unzips in a single abrupt step followed by further slight extension increases. ( b ) Typical unwinding event of AtRECQ2 on a 40 bp hairpin in the presence of ATP at a constant force of 10 pN. After slow hairpin unwinding an abrupt rezipping of the hairpin occurs followed by a resetting, that is, the reinititation of a new unwinding event (see sketches below). ( c ) Global unwinding pattern of AtRECQ2 on the 40 bp DNA hairpin under the same conditions as in b . (upper) Individual saw tooth-like events of similar size occur in a highly repetitive fashion. (lower). Periods of highly repetitive unwinding events are interspersed with periods of no activity. Full size image To observe unwinding of the hairpin by AtRECQ2, the force is set below F unzip and the enzyme is added in the presence of ATP. After a while characteristic events in which the DNA extension slowly but progressively increases (mean unwinding velocity of 8 bp s −1 , see below) can be observed ( Fig. 1b ). No DNA lengthening is observed when using AtRECQ2-K117M that carries a mutation in the Walker A motif and displays inhibited ATPase activity. This indicates that the observed events for the wt enzyme are due to DNA unwinding by AtRECQ2. When the full 40 bp are unwound, typically an abrupt resetting to a partially or fully closed hairpin state is observed. The slow unwinding followed by a very fast resetting is characteristic for AtRECQ2, independent of the DNA template length, the bp composition or the applied forces (see below). Individual unwinding events typically occur in a highly repetitive fashion ( Fig. 1c , upper graph) within confined time intervals ( Fig. 1c , lower graph), that is, bursts of many unwinding events are separated by long pauses. This strongly suggests that a single enzyme or enzyme-complex is responsible for the repetitive unwinding until it dissociates. The long pauses are then the time required for binding of the next enzyme or enzyme-complex. If a single enzyme-complex is responsible for the repetitive DNA unwinding, it remains, however, unclear how the fast reinitiation of unwinding is achieved, during which AtRECQ2 has to move quickly from the hairpin end-loop to the ssDNA initiation site at the closed hairpin. This cannot be explained by a remaining contact of the helicase with the 5′-end of the displaced strand as suggested for the RNA helicase NS3 (ref. 20 ). This would involve the extrusion of a ssDNA loop in disagreement with an average maximum increase in DNA length for DNA unwinding by AtRECQ2 corresponding to the fully opened hairpin of 83 nt ( Supplementary Fig. S1b ). Therefore, the enzyme has to move along the unwound DNA for reinitiation of unwinding. Loose DNA contacts on ssDNA in the absence of a DNA junction To gain insight into the reinitiation process, we studied the behaviour of AtRECQ2 on ssDNA, which it encounters, for example, after complete hairpin unwinding. For this, we used a 488 bp long hairpin construct. During DNA unwinding by the helicase, this hairpin is mechanically unzipped by applying a force F > F unzip , after which the helicase is left only with ssDNA ( Fig. 2a ). After a specified time τ open the force is reduced again ( F < F unzip ) and the hairpin rehybridizes until it encounters the enzyme. The change of the hairpin length from just before unzipping until just after rezipping is then attributed to the distance the helicase moved on ssDNA during τ open . To rule out that the observed changes in the hairpin length originate from dissociation and rebinding of different enzymes during τ open , periodic unzipping-rezipping cycles were performed independent of the presence of a helicase on the DNA ( Supplementary Fig. S2a ). 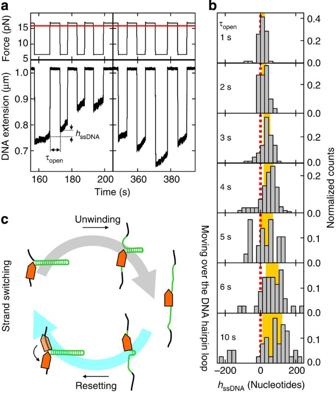Figure 2: Behaviour of AtRECQ2 on single-stranded DNA. (a) Measuring the distance AtRECQ2 moved on ssDNA by repetitive cycles of hairpin unzipping. A 488 bp long DNA hairpin (Funzip=15.8 pN, upper graph red solid line) is mechanically un- and rezipped by switching the force betweenF=6.6 pN (hairpin closed) andF=16.8 pN (hairpin open). At the low force, a slowly increasing DNA extension indicates hairpin unwinding by the helicase. Switching to the high force unzips the hairpin, seen as a sudden large increase of the DNA extension. The hairpin is kept open for the timeτopen, after which the force is lowered and the hairpin rezips until it encounters the helicase. The distance that the enzyme moved on the unzipped ssDNA (hssDNA) is then the difference of the hairpin lengths just after and just before hairpin re- and unzipping, respectively. (b) Histograms ofhssDNAfor increasingτopen(as given in the plots). The red dotted line indicateshssDNA=0. The yellow area indicates the region within the s.d. of the distribution around its mean. Only events for which AtRECQ2 did not reach the end of the hairpin were considered. (c) Model for repetitive DNA unwinding by AtRECQ2 of the 40 bp hairpin. After full unwinding of the DNA hairpin the enzyme becomes more loosely bound to ssDNA. After it moves over the hairpin loop, the rehybridizing hairpin pushes the helicase along the formerly displaced strand until the hairpin is closed. Subsequently the helicase switches back to the original tracking strand and initiates a new unwinding event. Figure 2: Behaviour of AtRECQ2 on single-stranded DNA. ( a ) Measuring the distance AtRECQ2 moved on ssDNA by repetitive cycles of hairpin unzipping. A 488 bp long DNA hairpin ( F unzip =15.8 pN, upper graph red solid line) is mechanically un- and rezipped by switching the force between F =6.6 pN (hairpin closed) and F =16.8 pN (hairpin open). At the low force, a slowly increasing DNA extension indicates hairpin unwinding by the helicase. Switching to the high force unzips the hairpin, seen as a sudden large increase of the DNA extension. The hairpin is kept open for the time τ open , after which the force is lowered and the hairpin rezips until it encounters the helicase. The distance that the enzyme moved on the unzipped ssDNA ( h ssDNA ) is then the difference of the hairpin lengths just after and just before hairpin re- and unzipping, respectively. ( b ) Histograms of h ssDNA for increasing τ open (as given in the plots). The red dotted line indicates h ssDNA =0. The yellow area indicates the region within the s.d. of the distribution around its mean. Only events for which AtRECQ2 did not reach the end of the hairpin were considered. ( c ) Model for repetitive DNA unwinding by AtRECQ2 of the 40 bp hairpin. After full unwinding of the DNA hairpin the enzyme becomes more loosely bound to ssDNA. After it moves over the hairpin loop, the rehybridizing hairpin pushes the helicase along the formerly displaced strand until the hairpin is closed. Subsequently the helicase switches back to the original tracking strand and initiates a new unwinding event. Full size image A unidirectional movement along the 3′–5′ direction of the enzyme along ssDNA would lead to only positive moved distances with respect to the hairpin unwinding direction [10] , [21] . In contrast, we observe in these unzipping experiments positive as well as negative distances moved on ssDNA, while the helicase always exclusively moves along the unwinding direction on the closed hairpin in these experiments ( Fig. 2a ). To reveal the origin of the negative distances, we systematically varied τ open . With increasing τ open , the mean of the distance distribution increases with 10 nt s −1 in agreement with unidirectional translocation on ssDNA ( Fig. 2b ; Supplementary Fig. S3a ). In addition, however, the variance of the distribution increases strongly ( Fig. 2b ; Supplementary Fig. S3b ), which is due to the negative distances and suggests an additional bidirectional, that is, diffusive, movement of the enzyme on ssDNA. The negative distances moved on ssDNA cannot be caused by the rezipping hairpin that may push the helicase backwards along its tracking strand. Such an event should cause a constant shift or variance increase of the distance distribution independent of τ open . Altogether, this suggests that AtRECQ2 is strongly bound to its tracking strand in presence of an unwinding fork, where it processively unwinds DNA. On ssDNA, however, it undergoes translocation as well as a slow diffusive motion ( Supplementary Fig. S3b ). Diffusion of proteins on ssDNA with similar diffusion constants has been previously observed for E. coli SSB [22] as well as for the cytosine deaminase APOBEC3G [23] . Translocation and diffusion are likely two distinct modes of movement on ssDNA between which AtRECQ2 alternates (see analysis of resetting events below). Sliding-based mechanism for the repetitive unwinding by AtRECQ2 From these observations, we hypothesize the following model for repetitive DNA unwinding by AtRECQ2 on the 40 bp hairpin ( Fig. 2c ): After binding to the closed hairpin, the helicase processively unwinds it following its tracking strand along the 3′–5′ direction. Once the hairpin is fully unwound, the helicase moves beyond the end-loop of the hairpin and adopts a more loosely bound conformation in which it further translocates or diffuses (slides). The hairpin then starts to rezip and pushes the sliding helicase along the previously displaced strand. A new unwinding event is then initiated when the helicase strand switches on the rezipped hairpin from the displaced to the tracking strand. This model is based on several assumptions: (i) during hairpin rezipping, the enzyme behaves as on ssDNA, hat is, it partially translocates and partially slides; (ii) the enzyme performs strand switches; (iii) the enzyme verifies the presence of the junction and senses how it is positioned with respect to the junction. This is important to allow the enzyme to processively unwind the hairpin along the tracking strand, but efficiently slide back along the formerly displaced strand. In the following, additional experimental evidence is provided to substantiate these assumptions. Resetting events display similar characteristics as AtRECQ2 on ssDNA In the majority of resetting events, the 40 bp hairpin rezips in a single fast step (83% of all events at 10 pN stretching force). The remaining events contain in addition to fast rezipping, stretches of much slower hairpin closure with similar velocities as unwinding (9.3±1 bp s −1 , Fig. 3a–c (ii)). Most likely this can be attributed to hairpin rewinding driven by translocation of the helicase along the previously displaced strand. Thus, there is coexistence of fast hairpin rezipping due to enzyme sliding and slow rewinding. This is similar to the enzyme behaviour on ssDNA and suggests that also there the enzyme switches between translocation and diffusion. 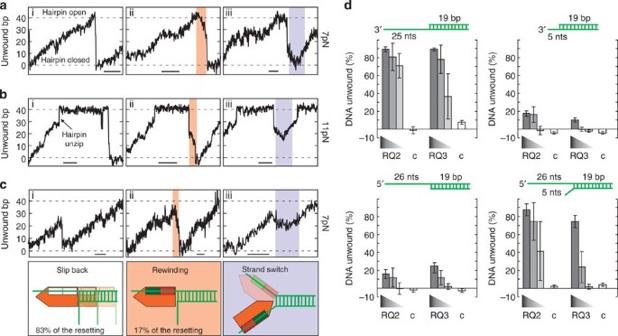Figure 3: Partial rewinding and direction reversals of AtRECQ2. (a–c) Selected unwinding events recorded on the 40 bp DNA hairpin. Dashed lines indicate the position of the fully closed and the fully open DNA hairpin. The scale bars indicate 1 s. The small roman numbers in the graphs correspond to the following types of resetting event as illustrated with sketches below the graphs: (i) continuous, abrupt hairpin rezipping; (ii) abrupt rezipping and partial slow rewinding; and (iii) direction reversals from rewinding to unwinding. In (a,b) events in which the hairpin is fully unwound, which were recorded at forces of 7 and 11 pN, respectively, are depicted. At the high force the hairpin spontaneously unzips shortly before full unwinding and may stay open for a longer period. Inc, incomplete unwinding events taken at 7 pN are shown. (d) Bulk unwinding experiments. Used DNA substrates are sketched above each graph. In all, 0.15 nM DNA was incubated with decreasing concentrations (as illustrated by the wedge symbol) of AtRECQ2 (18, 6 and 2 nM) or AtRECQ3 (25, 8 and 3 nM) and with 19 nM AtRECQ2-K117M or 18 nM AtRECQ3-K64M (indicated with c) in the presence of ATP. Reaction products were analysed by native gel electrophoreses and the amount of DNA unwinding determined. The error bars represent the s.d. of four individual measurements. nts, nucleotides. Figure 3: Partial rewinding and direction reversals of AtRECQ2. ( a – c ) Selected unwinding events recorded on the 40 bp DNA hairpin. Dashed lines indicate the position of the fully closed and the fully open DNA hairpin. The scale bars indicate 1 s. The small roman numbers in the graphs correspond to the following types of resetting event as illustrated with sketches below the graphs: (i) continuous, abrupt hairpin rezipping; (ii) abrupt rezipping and partial slow rewinding; and (iii) direction reversals from rewinding to unwinding. In ( a , b ) events in which the hairpin is fully unwound, which were recorded at forces of 7 and 11 pN, respectively, are depicted. At the high force the hairpin spontaneously unzips shortly before full unwinding and may stay open for a longer period. In c , incomplete unwinding events taken at 7 pN are shown. ( d ) Bulk unwinding experiments. Used DNA substrates are sketched above each graph. In all, 0.15 nM DNA was incubated with decreasing concentrations (as illustrated by the wedge symbol) of AtRECQ2 (18, 6 and 2 nM) or AtRECQ3 (25, 8 and 3 nM) and with 19 nM AtRECQ2-K117M or 18 nM AtRECQ3-K64M (indicated with c) in the presence of ATP. Reaction products were analysed by native gel electrophoreses and the amount of DNA unwinding determined. The error bars represent the s.d. of four individual measurements. nts, nucleotides. Full size image Strand switching by AtRECQ2 If the proposed strand switching occurs, sudden direction changes from hairpin rewinding to unwinding and potentially also from unwinding towards rewinding should be observable. The majority of unwinding events is terminated by abrupt rezipping, where such direction changes cannot be directly observed. However, for the events that display rewinding, directional changes can be frequently found (column (iii) in Fig. 3a–c ). Direction reversals occur after full rewinding of the hairpin ( Fig. 3a ), during rewinding at the still partially open hairpin ( Fig. 3b ) or during unwinding at the not yet fully open hairpin ( Fig. 3c ). This demonstrates the capability of the enzyme to strand switch, if direct translocation direction reversals are excluded. SF1 helicases translocate along the 3′–5′ (SF1A) or the 5′–3′ (SF1B) direction, but bind ssDNA in the same orientation with respect to the N- and the C-terminal RecA-like domains [24] , [25] , [26] , [27] , [28] , [29] . A different translocation direction is achieved by modulating the nucleotide-dependent affinities of the two RecA-like domains to ssDNA in an inverted order. An allosteric affinity change leading to a direct direction reversal seems then to be too complicated. To obtain further evidence for strand switching, we carried out bulk-solution strand displacement assays. If strand switching occurs, a 5′ overhang on a duplex DNA molecule, should then be able to assist loading of the helicase onto the neighbouring 3′ end. To test this hypothesis, we prepared two dsDNA substrates, one with a 25 and the other with 5 nt 3′ overhang. Although the former molecule is efficiently unwound by AtRECQ2, unwinding on the latter overhang is almost entirely impeded ( Fig. 3d ), as the helicase does not efficiently load onto such a short overhang. Unwinding of a DNA duplex with a 26 nt long 5′ overhang is also inefficient ( Fig. 3e ) due to the 3′–5′ directionality of the helicase. However, on a substrate that has in addition to a short 5 nt long 3′ overhang a 26 nt long 5′ overhang, efficient unwinding is restored, which is in agreement with a facilitation of the helicase loading process by strand switching ( Fig. 3e ). Previously, it has been shown that RecQ helicases, for example, HsWRN, preferentially bind to forked DNA substrates [30] . AtRECQ2 interacts with both DNA strands at the unwinding junction For the junction sensing according to our model, AtRECQ2 should make contacts to its tracking strand as well as the displaced strand being already ssDNA or still within the DNA duplex at the junction. To verify contacts to both strands we measured the necessary force to unzip the DNA hairpin in the presence of the enzyme using the 488 bp long hairpin. In the absence of enzyme, this hairpin becomes unzipped at forces ≥16 pN. In experiments where the force is changed from 10.4 pN to 18 pN, it opens in 100% of all unzipping attempts ( Fig. 4a ), and still in 88% of all attempts for force switches from 10.4–16 pN. 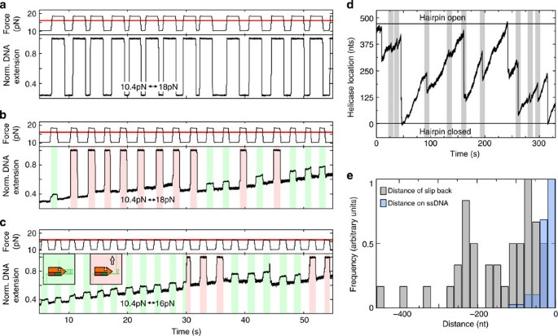Figure 4: Clamping of the unwinding fork by AtRECQ2. (a) Repetitive mechanical unzipping of a 488 bp long hairpin in absence of AtRECQ2 by switching the force between 10.4 and 18 pN. The red solid line in the upper graph indicates the unzipping force. (b) Repetitive force switching between 10.4 and 18 pN for the hairpin inaduring unwinding by AtRECQ2. White areas indicate periods of low force. Coloured areas represent periods at high force during which the hairpin fully unzips (red) or remains fully closed (green). (c) Same experiment as inbfor force switches between 10.4 and 16 pN. (d) DNA unwinding of the 488 bp long hairpin by AtRECQ2 at 10 pN force. The positions of the fully closed and the fully opened DNA hairpin are indicated with black solid lines. Abrupt rezipping events starting before the full hairpin is unwound and ending before it is fully closed are indicated with light grey boxes. (e) Histogram of the distances of abrupt rezipping events for which the hairpin does not fully close (shown in grey, see D for details). For comparison, a histogram of the negative moved distances on ssDNA (hssDNA, from the experiments shown inFig. 2afor hairpin opening times <3 s) is shown in blue. nt, nucleotide. Figure 4: Clamping of the unwinding fork by AtRECQ2. ( a ) Repetitive mechanical unzipping of a 488 bp long hairpin in absence of AtRECQ2 by switching the force between 10.4 and 18 pN. The red solid line in the upper graph indicates the unzipping force. ( b ) Repetitive force switching between 10.4 and 18 pN for the hairpin in a during unwinding by AtRECQ2. White areas indicate periods of low force. Coloured areas represent periods at high force during which the hairpin fully unzips (red) or remains fully closed (green). ( c ) Same experiment as in b for force switches between 10.4 and 16 pN. ( d ) DNA unwinding of the 488 bp long hairpin by AtRECQ2 at 10 pN force. The positions of the fully closed and the fully opened DNA hairpin are indicated with black solid lines. Abrupt rezipping events starting before the full hairpin is unwound and ending before it is fully closed are indicated with light grey boxes. ( e ) Histogram of the distances of abrupt rezipping events for which the hairpin does not fully close (shown in grey, see D for details). For comparison, a histogram of the negative moved distances on ssDNA ( h ssDNA , from the experiments shown in Fig. 2a for hairpin opening times <3 s) is shown in blue. nt, nucleotide. Full size image This changes in the presence of AtRECQ2. For force switches to 18 pN, carried out after initiation of unwinding by the helicase the hairpin unzips only in 65% of the attempts ( Fig. 4b ). For the remaining 35%, the applied force stretched the dsDNA spacer and the already unwound ssDNA, while the hairpin was further unwound by the helicase. For force switches to 16 pN the hairpin remained closed in even 80% of all attempts ( Fig. 4c ). Thus, AtRECQ2 interacts with both DNA strands of the hairpin and clamps the two strands together. Further verification of the preferred binding of AtRECQ2 to the junction is obtained from competition DNA-unwinding assays ( Supplementary Fig. S4 ). The observed clamping of the unwinding fork by AtRECQ2 is also in agreement with the low force but strong DNA sequence dependence of the unwinding velocity ( Supplementary Fig. S5 ). For other SF2 helicases also a low force dependence and a more [31] or less [21] strong sequence dependence was found. This is in contrast to hexameric helicases studied so far that exhibit both a strong force and sequence dependence [10] , [11] , [21] , [32] . In addition to the interaction with both strands at the unwinding fork, AtRECQ2 should also sense the location of the junction either being in front or behind of the enzyme with respect to the unwinding direction. Evidence for such sensing is provided by analysing the length of resetting events on the 40 bp and the 488 bp long hairpin construct. Assuming that after unwinding the double-stranded region of the 40 bp hairpin construct the enzyme is passing the end-loop and translocating on the displaced strand, it will be in a different orientation to the rehybridizing hairpin than during unwinding ( Fig. 2c ). The fork will be behind the enzyme. After complete unwinding, a mean distance of spontaneous resetting events ( Fig. 1 ) of 33 bp is observed. In contrast, during the unzipping experiments that measured the movement of AtRECQ2 on ssDNA, the enzyme follows the tracking strand and the junction is located in front of the enzyme. Here, we obtain an average negatively moved distance on ssDNA of only 18 bp for hairpin opening times of ≤3 s ( Figs. 2b , 4e ). In addition, there is no indication that the rezipping hairpin can slide the enzyme backwards against the tracking direction (see above), supporting the idea that during the fast resetting events the fork may be located behind the enzyme. Spontaneously occurring resetting events can also be observed for the 488 bp hairpin construct. Most of these fast resetting events occur before the hairpin is fully unwound and are, with an average length of 140 bp ( Fig. 4d ), much larger than the negatively moved distances on ssDNA in the unzipping experiments. This again suggests that for the fast resetting events, the fork is behind the enzyme, which requires that the enzyme switches strands during hairpin unwinding and in this way triggers the long spontaneous resetting events. It is then pushed back by the rezipping hairpin that comes from behind. Thus, the presence of two different length scales for spontaneous resetting on the one hand and sliding on ssDNA on the other hand is in agreement with a directional sensing of the DNA junction. However, we note that direct backsliding with the junction being in front of the enzyme cannot be ruled out by the presented data. AtRECQ3 displays a different unwinding behaviour To investigate whether the observed unwinding–resetting cycles of AtRECQ2 are general characteristics of RecQ helicases from A. thaliana , we carried out similar experiments with AtRECQ3. We measured DNA unwinding by AtRECQ3 using the 488 bp hairpin. Strikingly, unwinding events of AtRECQ3 are very different compared with AtRECQ2 under otherwise same conditions ( Fig. 5a ). DNA unwinding is always followed by DNA rewinding at equal velocity ( Supplementary Fig. S6a ). Fast rezipping events as seen for AtRECQ2 were never observed. When using AtRECQ3 K64M [8] with a mutation in the Walker A motif, no unwinding was detected. AtRECQ3 was also by far not able to unwind the full hairpin. Unwinding terminated after only few tens of bps ( Fig. 5a ) followed by a direction reversal. Similarly to AtRECQ2, the unwinding events for AtRECQ3 occurred in a highly repetitive manner, where long periods of activity and no activity were alternating ( Fig. 5a ). This indicates that the repetitive cycles of unwinding and rewinding are caused by a single enzyme-complex. In agreement with this, the average time between individual events of about 3 s remains within error unchanged for a 20-fold lower enzyme concentration, but the pauses between the bursts of activity become markedly longer. 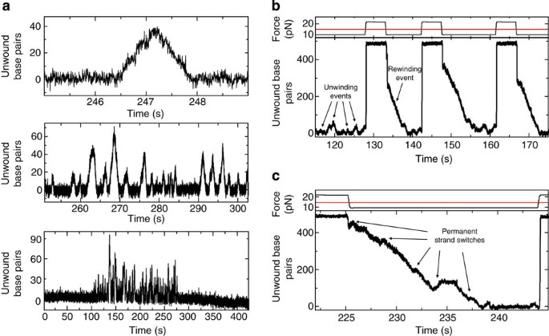Figure 5: DNA unwinding and rewinding by AtRECQ3. (a) Unwinding pattern of AtRECQ3 on the 488 bp DNA hairpin in the presence of ATP at constant force of 10 pN. (upper) Slow DNA unwinding is always followed by slow DNA rewinding. (middle) Individual unwinding–rewinding events of similar extent occur in a highly repetitive fashion. The AtRECQ3 catalysed DNA unwinding is much shorter than the full-length of the hairpin. (lower) Periods of highly repetitive unwinding events are interspersed with periods of no activity. (b) Unzipping and rezipping the 488 bp DNA hairpin during activity of AtRECQ3. Corresponding force switches are shown in the top graph. The red line indicatesFunzip. In contrast to the very short unwinding distances found for AtRECQ3, the DNA hairpin is processively rewound over hundreds of bp (events indicated by arrows). (c) Enlarged view into an individual rewinding event reveals permanent direction reversals from rewinding to unwinding and back to rewinding. Figure 5: DNA unwinding and rewinding by AtRECQ3. ( a ) Unwinding pattern of AtRECQ3 on the 488 bp DNA hairpin in the presence of ATP at constant force of 10 pN. (upper) Slow DNA unwinding is always followed by slow DNA rewinding. (middle) Individual unwinding–rewinding events of similar extent occur in a highly repetitive fashion. The AtRECQ3 catalysed DNA unwinding is much shorter than the full-length of the hairpin. (lower) Periods of highly repetitive unwinding events are interspersed with periods of no activity. ( b ) Unzipping and rezipping the 488 bp DNA hairpin during activity of AtRECQ3. Corresponding force switches are shown in the top graph. The red line indicates F unzip . In contrast to the very short unwinding distances found for AtRECQ3, the DNA hairpin is processively rewound over hundreds of bp (events indicated by arrows). ( c ) Enlarged view into an individual rewinding event reveals permanent direction reversals from rewinding to unwinding and back to rewinding. Full size image For the repetitive unwinding–rewinding cycles we propose that AtRECQ3 unwinds the DNA hairpin by tracking along the 3′–5′ direction. After few tens of bps, it switches to the displaced strand, tracks on it along the 3′–5′ direction and the reannealing of the hairpin behind the helicase leads to the apparent slow hairpin ‘rewinding’. A new unwinding event is then started after a further strand switch. As for AtRECQ2, the cycle for repetitive events of AtRECQ3 relies on repeated strand switches. We also performed experiments where the DNA hairpin is mechanically unzipped while the enzyme is unwinding or rewinding it. In contrast to AtRECQ2, AtRECQ3 is a bona fide ssDNA translocase with no backward movement on ssDNA compared with its original winding direction ( Supplementary Fig. S7 ). Strikingly, when the hairpin was kept open for an extended period of time, AtRECQ3 started immediate rewinding of the DNA hairpin after the force was lowered below F unzip ( Fig. 5b ). The opposite is found for AtRECQ2, which always unwinds the DNA after rezipping. The rewinding process of AtRECQ3 is much more processive than the corresponding unwinding. This is a new helicase activity that has only one very recent precedent [33] . A closer look into the individual rewinding events shows that during rewinding, the helicase switches back to unwinding from time to time ( Fig. 5c ). The unwinding is again not very processive and rewinding is recommenced after few tens of bp, providing an overall long and processive DNA rewinding. We also verified that the rewinding activity of AtRECQ3 has a strict requirement for ATP hydrolysis ( Supplementary Fig. S8 ). Furthermore, binding specificities are in line with rewinding ( Supplementary Fig. S4 ) and no indication of clamping of the DNA junction was found in unzipping experiments. In summary, we show here that both AtRECQ2 and AtRECQ3 exhibit highly repetitive DNA unwinding activity, in which a single enzyme-complex maintains its contact to the DNA junction to reinitiate a large number of events. Together with the observed repetitive DNA unwinding for HsBLM [16] , this suggests that repetitive DNA unwinding is a widespread activity of RecQ helicases. Most interestingly AtRECQ2 and AtRECQ3 show largely antagonistic activities. Although AtRECQ2 predominantly orients itself to unwind DNA, AtRECQ3 turns around after unwinding short DNA stretches, to predominantly rewind DNA. For both helicases strand switches seem to be crucial for the repetitive unwinding. With this, we can sketch a unified model for the repetitive DNA unwinding–rewinding/resetting cycles of both helicases ( Fig. 6 ). Intriguingly, this model provides a simple way to reverse the overall unwinding direction although still using the same mechanism. The net average unwinding distance is determined by the frequencies of the strand switches from unwinding to rewinding, (C in Fig. 6 ) versus rewinding to unwinding, (E in Fig. 6 ) as well as the ratio of the unwinding versus the rewinding/rezipping velocities. For AtRECQ3, the unwinding and the rewinding velocities are equal ( Supplementary Fig. S6a ), but it switches more rapidly from unwinding to rewinding than vice versa (compare the mean unwinding time versus the mean time between unwinding events in Supplementary Fig. S6c,d ). This leads to an effective DNA rewinding for AtRECQ3. In contrast, for AtRECQ2 the frequency of strand switching from unwinding to rewinding is much lower than the frequently observed instantaneous switches from rezipping to unwinding, which can even occur during the slippage process ( Fig. 4d ). This way, AtRECQ2 spends most of the time unwinding DNA. As the slippage is, however, much faster than the slow unwinding, the unwinding distance is also limited and can be controlled by inhibiting strand switching, for example, with external force ( Fig. 4e ; Supplementary Fig. S9 ). For AtRECQ2, we furthermore provide evidence that it can sense the presence of the unwinding fork (possibly even relative to its own orientation, see Fig. 4d ) most likely due to its interaction with both DNA strands of the DNA junction ( Fig. 4a–c , Supplementary Fig. S4 ), which is probably the requirement for such a sensing. 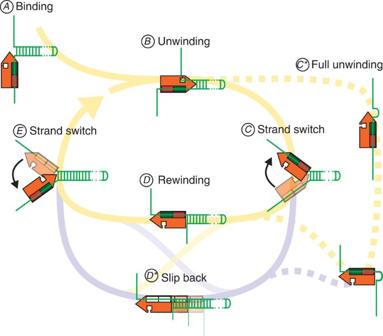Figure 6: Unified model for repetitive DNA unwinding by AtRECQ2 and AtRECQ3. The helicase is sketched in orange with its tip representing the RecQ-C-terminal domain, where the bp opening is catalysed. The red and green rectangles represent the two RecA-like domains. Uncoloured RecA-like domains symbolize low affinity to the ssDNA during sliding. During unwinding, the DNA junction is clamped symbolized by the enzyme-captured displaced strand. After binding to a 3′ overhang (A), the helicases start to processively unwind the duplex DNA by tracking along the 3′–5′ direction (B). The unwinding reaction stops either due to a spontaneous strand switch from the tracking to the displaced strand (C) or due to the full unwinding of the DNA hairpin (C*). The helicases may then continue to slowly translocate along the formerly displaced strand (D). This leads to slow rewinding of the hairpin, as it reanneals behind the helicase. Alternatively, AtRECQ2 may also rapidly slip back along the displaced strand while being pushed by the reannealing hairpin (D*). As shown above, AtRECQ2 is not only translocating on ssDNA but can in contrast to AtRECQ3 adopt a weaker bound diffusive state (Fig. 2), which supports the slippage. After rewinding or, respectively, resetting, the enzyme switches back from the formerly displaced (the actual tracking strand) to the original tracking strand (E) and reinitiates a new unwinding cycle. Figure 6: Unified model for repetitive DNA unwinding by AtRECQ2 and AtRECQ3. The helicase is sketched in orange with its tip representing the RecQ-C-terminal domain, where the bp opening is catalysed. The red and green rectangles represent the two RecA-like domains. Uncoloured RecA-like domains symbolize low affinity to the ssDNA during sliding. During unwinding, the DNA junction is clamped symbolized by the enzyme-captured displaced strand. After binding to a 3′ overhang (A), the helicases start to processively unwind the duplex DNA by tracking along the 3′–5′ direction (B). The unwinding reaction stops either due to a spontaneous strand switch from the tracking to the displaced strand (C) or due to the full unwinding of the DNA hairpin (C*). The helicases may then continue to slowly translocate along the formerly displaced strand (D). This leads to slow rewinding of the hairpin, as it reanneals behind the helicase. Alternatively, AtRECQ2 may also rapidly slip back along the displaced strand while being pushed by the reannealing hairpin (D*). As shown above, AtRECQ2 is not only translocating on ssDNA but can in contrast to AtRECQ3 adopt a weaker bound diffusive state ( Fig. 2 ), which supports the slippage. After rewinding or, respectively, resetting, the enzyme switches back from the formerly displaced (the actual tracking strand) to the original tracking strand (E) and reinitiates a new unwinding cycle. Full size image The mechanism of the strand switching still remains elusive. It could be achieved if one additional enzyme domain remains in contact to the DNA duplex part of the junction and allows the switching and repositioning of the two RecA-like domains. An idea of how this may be achieved is provided by a recent study of the SF1 enzyme PcrA [17] . For this enzyme, the turning of an anchor domain, attached to the dsDNA at the junction, allowed switching the ssDNA along which the enzyme translocats thus turning the enzyme from a helicase into a ‘reelicase’. For RecQ helicases such an anchor domain has not yet been identified. For HsBLM, it has been suggested that the RecQ-C-terminal and the helicase and RNaseD C-terminal (HRDC) domain may provide the required anchor for strand switching [16] , [34] , [35] . In agreement with this idea, a crystal structure of HsRECQ1 shows that the RecQ-C-terminal domain makes extensive contacts to the dsDNA at the fork [36] . Notably, AtRECQ3 does not have an HRDC domain and possesses of the RecQ-C-terminal domain only the conserved Zn-binding domain, while a pronounced winged helix motif is lacking [8] . A recent biochemical study showed that HsBLM that was truncated after the Zn-binding domain unwinds dsDNA similarly to the wild-type enzyme [37] . Therefore, it is possible that the winged helix and the HRDC domain are responsible for recognizing other target structures, such as Holliday junctions, while already the core of the enzyme including the two RecA-like domains and the Zn-binding domain may support the strand switching. Alternatively, as oligomerization for some RecQ helicases is found [38] , anti-parallel dimers of two RecQ monomers may also drive the strand switching that leads to the direction reversals [39] . We think that the antagonistic DNA-unwinding activities of AtRECQ2 and AtRECQ3 are important for their functions in vivo . AtRECQ2 may keep short stretches of DNA ends constantly open and thus provide access for other enzymes during repair processes, while AtRECQ3 may help to (re)hybridize complementary DNA strands by removing secondary structures or single-strand binding proteins such as RPA and RAD51. The preference of AtRECQ3 to move away from the fork may also explain its preference to unwind the lagging strand of a synthetic stalled replication fork [8] . It may be that other RecQ helicases are more efficient DNA rewinders rather than unwinders. A promising candidate would be HsRECQ5β that disrupts RAD51 filament formation [40] , [41] . It has a similar unwinding preference on synthetic stalled replication forks as AtRECQ3 (ref. 42 ). For HsRECQ5β, a BRC variant motif was identified recently. Those amino acids are involved in RAD51 interaction [43] . In AtRECQ3, we find a region adjacent to the Zn-finger ( F I T S SN N K T N EGQYSEFWNRNEDGSNS), which has similarities to the BRC3 repeat of AtBRCA2 ( F Q T A SN K K V N VS SAGLARAKALLG) [44] . Thus, it is tempting to speculate that AtRECQ3 has a similar role as HsRECQ5β. In general, our unifying model for AtRECQ2 and AtRECQ3 is attractive to explain how RecQ helicases can achieve opposite effects in vivo , by differentially changing the strand switching activities in the repetitive cycle. In addition, the force sensitivity of the strand switching ( Supplementary Fig. S9 ) may provide a way to control the activity of the helicases, as enzymes that bind to the displaced strand may have a similar force effect on the junction. Enzymes and DNA AtRECQ2 and AtRECQ3 were purified as described [7] , [8] , [45] . Briefly, they were purified by Ni-IMAC (C-terminal 6xHis-tag) followed by calmodulin affinity chromatography (N-terminal calmodulin-binding peptide). DNA substrates for single-molecule experiments ( Supplementary Fig. S1 ) contained a hairpin of either 40, 90 or 488 bp length that carried a biotin modification at its 5′-ends (separated by a short ssDNA spacer) to allow attachment to the streptavidin-coated magnetic bead. At its 3′-end, the hairpin carried a ssDNA initiation site for the helicase followed by a long dsDNA spacer and a 600 bp long digoxigenin-modified handle that supports attachment to the anti-digoxigenin-coated surface of the fluidic cell of the setup. Hairpin substrates were prepared by ligating the hairpin, the dsDNA spacer and the dsDNA handle through suitable overhangs [46] . Spacers and handles were made by PCR in, respectively, absence and presence of digoxigenin-labeled dUTPs [47] . Short DNA hairpins (40, 90 bp) were prepared by annealing synthetic DNA oligomers, with one of them being biotinylated on the 5′-end, followed by ligation [48] . The long DNA hairpin was prepared by ligating two dsDNA PCR fragments, each consisting of a 488 bp long homologous region followed by a shorter heterologous region, at their homologous ends. One fragment carried a 5′-biotin at its heterologous end. Subsequently, the non-biotinylated DNA strand of the ligation product was digested with lambda exonuclease (NEB), resulting into folding of a 488 bp hairpin with shorter ssDNA tails. Bulk strand displacement assay The bulk strand displacement assay was carried out as described [7] , [8] , [45] . The sequences of the oligonucleotides were published in a characterization of HsWRN [30] . As for HsWRN, the reaction was carried out with an excess of Mg 2+ -ions (4.5 mM MgCl 2 and 1.8 mM ATP). Incubation was at 37 °C for 20 min. Magnetic tweezers experiments The magnetic tweezers setup has previously been described in detail [19] , [49] . The position of the magnetic bead above the surface and thus the DNA length of the hairpin is determined by videomicroscopy with nanometre accuracy [19] , [50] . Images were acquired at a rate of 300 Hz. The DNA hairpin constructs were incubated with streptavidin-coated magnetic beads (Myone, Invitrogen) and subsequently attached to the anti-digoxigenin-coated surface of the fluidic cell in which the experiments were carried out. After calibrating the magnetic forces acting on the construct, AtRecQ2 or AtRecQ3 (8 nM) were added in 40 mM TrisAcetate (pH 8), 50 mM K-Acetate, 6 mM DTT, 50 μg ml −1 BSA, 1.8 mM ATP and 1.8 mM MgCl 2 . All experiments were performed at room temperature. The DNA extension at a certain force was converted into bps by assuming full unwinding of the hairpin for the highest events ( Supplementary Fig. S1 ). How to cite this article: Klaue, D. et al . Fork sensing and strand switching control antagonistic activities of RecQ helicases. Nat. Commun. 4:2024 doi: 10.1038/ncomms3024 (2013).